Growth of non-phototrophic microorganisms using solar energy through mineral photocatalysis Phototrophy and chemotrophy are two dominant modes of microbial metabolism. To date, non-phototrophic microorganisms have been excluded from the solar light-centered phototrophic metabolism. Here we report a pathway that demonstrates a role of light in non-phototrophic microbial activity. In lab simulations, visible light-excited photoelectrons from metal oxide, metal sulfide, and iron oxide stimulated the growth of chemoautotrophic and heterotrophic bacteria. The measured bacterial growth was dependent on light wavelength and intensity, and the growth pattern matched the light absorption spectra of the minerals. The photon-to-biomass conversion efficiency was in the range of 0.13–1.90‰. Similar observations were obtained in a natural soil sample containing both bacteria and semiconducting minerals. Results from this study provide evidence for a newly identified, but possibly long-existing pathway, in which the metabolisms and growth of non-phototrophic bacteria can be stimulated by solar light through photocatalysis of semiconducting minerals. Photoautotrophy was once believed to be the ultimate energy-harvesting pathway for all living organisms on Earth until the discovery of chemoautotrophy, in which organisms harness chemical energy for growth [1] . Chemoautotrophs synthesize biomass from carbon dioxide (CO 2 ), and gain chemical energy from oxidation of inorganic compounds such as hydrogen gas (H 2 ), ammonium (NH 4 + ), nitrite (NO 2 − ), reduced sulfur compounds, and Fe 2+ (refs 2 , 3 , 4 ). Organotrophic organisms rely on organic carbon synthesized from either phototrophs or chemoautotrophs. Non-phototrophic organisms such as chemoautotrophs and heterotrophs are excluded from the realm of the solar light-dependent metabolism, owing to their lack of photosensitive cellular compounds. Nonetheless, this deficiency does not necessarily exclude the possibility that these organisms can directly or indirectly derive energy from sunlight through inorganic mediators such as semiconducting minerals. Similar to the important role of metals and metal-containing minerals in the evolution and metabolism of phototrophic life cycles [5] , [6] , [7] , [8] , [9] , minerals may be important in delivering solar energy to non-phototrophic organisms. Common semiconducting minerals, such as rutile (TiO 2 ), sphalerite (ZnS) and goethite (FeOOH), are solar responsive photocatalysts in nature [10] , [11] , [12] . When the incident light energy is greater than the bandgap between the valence band and the conduction band of these minerals, photoelectron-hole pairs can be generated and redox reactions are triggered with the release of energy. This form of energy, although indirectly, may be harvested by non-phototrophic microorganisms. In this study, we provide evidence in favour of a novel pathway, in which solar energy is converted to chemical energy by photocatalysis of semiconducting minerals to support and stimulate the growth of non-phototrophic microorganisms, and help shape microbial communities in nature. Under light irradiation, photocatalysis of semiconducting minerals rutile, sphalerite, and goethite produced photoelectrons that supported the growth of representative non-phototrophic microorganisms including chemoautotrophic and acidophilic Acidithiobacillus ferrooxidans , heterotrophic Alcaligenes faecalis , and a natural soil microbial community. Bacterial growth pattern was dependent on light wavelength and intensity, and closely matched the light absorption spectra of the minerals. The calculated photon-to-biomass conversion efficiency suggests that the light-induced and mineral-mediated pathway is probably less efficient than photosynthesis. Growth of A . ferrooxidans on photoelectrons A model experimental system consists of a P- (photocatalytic) and a C- (chemotrophic) chamber ( Fig. 1 ). This dual-chambered design isolates photocatalysis in the P-chamber from microbial metabolism in the C-chamber and allows the measurement of current density and the calculation of the photon-biomass conversion efficiency. The P-chamber consists of a graphite electrode coated with one of the three semiconducting minerals, that is, rutile, sphalerite, or goethite. On irradiation by simulated solar energy (a Xe lamp), pairs of negatively charged electrons and positively charged holes are generated from the semiconducting mineral. The electrons are excited from the valence band to the conduction band, leaving the holes in the valence band. A reductant (ascorbic acid) is used to scavenge positively charged holes in the P-chamber. The photoelectrons are then transferred to the C-chamber through an externally connected wire to support the growth of A. ferrooxidans , a chemoautotrophic and acidophilic bacterium. This bacterium was chosen in this study for its known ability to derive energy through the oxidation of Fe 2+ . 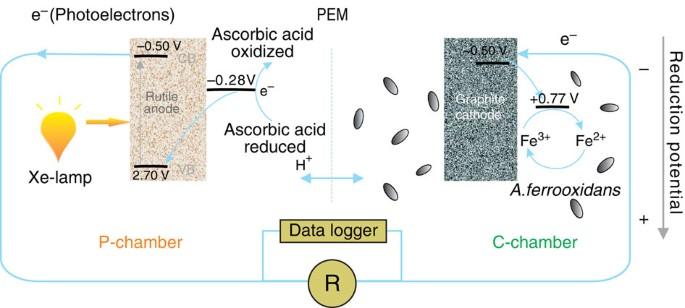Figure 1: A schematic diagram of the experimental system. The system consists of two chambers of 350 ml. each in size. The P-Chamber contains rutile or other semiconducting minerals (anode). On irradiation by a Xe lamp, the electrons are excited from the valence band (VB) with a reduction potential of 2.70 V to the conduction band (CB) with a reduction band of −0.50 V, whereas the positively-charged holes remain in the valence band. The holes were neutralized by the chemical reductant ascorbic acid. The redox couple of the reduced and oxidized ascorbic acid has a reduction potential of −0.28 V (ref.13); thus, the transfer of electrons from ascorbic acid to the valence band of rutile is a spontaneous process. The photoelectrons are transferred to the C-chamber through an externally connected wire, and the resulting current is determined by measuring the voltage through a 1,000 Ω external resistor using a data logger (ADC-16, Pico Technologies, UK). The electrons in the C-Chamber are captured by oxidants such as Fe3+that is produced by oxidation of Fe2+byA. ferrooxidans. This electron capture process is spontaneous because the reduction potential of graphite (slightly more positive than −0.50 V owing to the potential drop across the resistor) is more negative than the reduction potential of Fe3+/Fe2+at pH 2 (0.77 V). The proton exchange membrane (PEM) is used to allow exchange of protons across it to achieve charge balance between the two chambers. Figure 1: A schematic diagram of the experimental system. The system consists of two chambers of 350 ml. each in size. The P-Chamber contains rutile or other semiconducting minerals (anode). On irradiation by a Xe lamp, the electrons are excited from the valence band (VB) with a reduction potential of 2.70 V to the conduction band (CB) with a reduction band of −0.50 V, whereas the positively-charged holes remain in the valence band. The holes were neutralized by the chemical reductant ascorbic acid. The redox couple of the reduced and oxidized ascorbic acid has a reduction potential of −0.28 V (ref. 13 ); thus, the transfer of electrons from ascorbic acid to the valence band of rutile is a spontaneous process. The photoelectrons are transferred to the C-chamber through an externally connected wire, and the resulting current is determined by measuring the voltage through a 1,000 Ω external resistor using a data logger (ADC-16, Pico Technologies, UK). The electrons in the C-Chamber are captured by oxidants such as Fe 3+ that is produced by oxidation of Fe 2+ by A. ferrooxidans . This electron capture process is spontaneous because the reduction potential of graphite (slightly more positive than −0.50 V owing to the potential drop across the resistor) is more negative than the reduction potential of Fe 3+ /Fe 2+ at pH 2 (0.77 V). The proton exchange membrane (PEM) is used to allow exchange of protons across it to achieve charge balance between the two chambers. Full size image Two experiments were performed to demonstrate the light-induced growth of A. ferrooxidans . The first experiment was primarily designed to test the role of rutile photocatalysis in cell growth. Generation of photoelectrons from rutile on irradiation by a simulated sunlight source (visible light, continuous wavelength, 380–760 nm) was demonstrated by time-course production of Fe 2+ (green diamond, Fig. 2a ) in a bacteria-free and Fe 2+ -free m9K medium (see Methods for its complete composition). When bacteria were added to the C-chamber but without visible light in the P-chamber (that is, under the dark condition), cell concentration increased from 3.5×10 5 cells ml −1 at time zero to 3.6×10 7 cells ml −1 in 4 days (orange stars, Fig. 2a ) using the released energy from the oxidation of Fe 2+ initially present in the m9K medium (7,500 mg l −1 Fe 2+ ) (green stars, Fig. 2a ). When the graphite anode in the P-chamber was not coated with rutile (rutile-free), visible light could not produce any photoelectrons, and cell growth solely depended on the energy from the oxidation of Fe 2+ initially present in the m9K medium. Rapid cell growth (orange squares, Fig. 2a ) corresponded to rapid oxidation of Fe 2+ (green squares, Fig. 2a ) between day 1 and day 2.5, but the cell growth rate quickly decreased because of depletion of the medium-Fe 2+ to a negligible level. 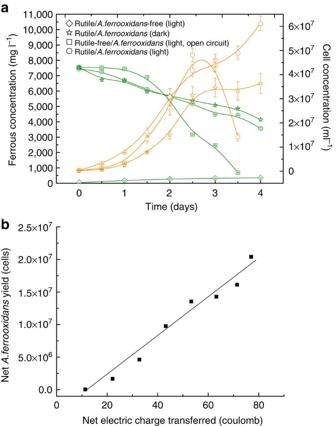Figure 2: Relationship betweenA. ferrooxidansgrowth and Fe2+concentration and electric charge transfer. (a) Time-course changes of Fe2+(green) andA. ferrooxidansconcentrations (orange) using rutile as a semiconducting mineral under different treatments. The P-chamber was either in the dark or irradiated with visible light (continuous wavelength 380–760 nm and ~13.5 mW cm−2). The cathode electrolyte is either the m9K medium (experiments withA.ferrooxidans) or Fe2+-free m9K medium (A.ferrooxidans-free experiment). The Fe2+-free m9K medium was made by replacing 41.7 g l−1FeSO4·7H2O with 6.1 g l−1FeCl3(equivalent to 2.1 g l−1Fe3+conc.). The slightly lower Fe2+concentration at time zero (that is, 7,500 mg l−1) than the expected value from 41.7 g l−1FeSO4·7H2O (Fe2+8382 mg l−1) for the treatments withA.ferrooxidanswas probably due to oxidation of Fe2+and precipitation of ferric oxide. The difference in cell concentration between the rutile-free reaction (rutile-free/A.ferrooxidans(light, open circuit)) and the rutile-catalysed process (rutile/A.ferrooxidans(light)) is about fivefold, and this difference is reproducible from multiple experiments. Ascorbic acid was used in all these treatments for the sole purpose of quenching positively charged holes remaining in the valence band of rutile. The role of ascorbic acid in promoting bacterial growth was expected to be minimal, as bacterial growth was not stimulated beyond that by the amount of Fe2+initially present in the m9K medium for the 'open-circuit' and dark controls. Even if there was any effect, this effect would have been present in all treatments and should not affect the relative comparison between them. (b) A significant positive correlation between the net growth ofA. ferrooxidansin the reactor and net electric charge transferred from the P-chamber to the C-chamber (Pvalue <0.001). Figure 2: Relationship between A. ferrooxidans growth and Fe 2+ concentration and electric charge transfer. ( a ) Time-course changes of Fe 2+ (green) and A. ferrooxidans concentrations (orange) using rutile as a semiconducting mineral under different treatments. The P-chamber was either in the dark or irradiated with visible light (continuous wavelength 380–760 nm and ~13.5 mW cm −2 ). The cathode electrolyte is either the m9K medium (experiments with A.ferrooxidans ) or Fe 2+ -free m9K medium ( A.ferrooxidans -free experiment). The Fe 2+ -free m9K medium was made by replacing 41.7 g l −1 FeSO 4 ·7H 2 O with 6.1 g l −1 FeCl 3 (equivalent to 2.1 g l −1 Fe 3+ conc.). The slightly lower Fe 2+ concentration at time zero (that is, 7,500 mg l −1 ) than the expected value from 41.7 g l −1 FeSO 4 ·7H 2 O (Fe 2+ 8382 mg l −1 ) for the treatments with A.ferrooxidans was probably due to oxidation of Fe 2+ and precipitation of ferric oxide. The difference in cell concentration between the rutile-free reaction (rutile-free/ A.ferrooxidans (light, open circuit)) and the rutile-catalysed process (rutile/ A.ferrooxidans (light)) is about fivefold, and this difference is reproducible from multiple experiments. Ascorbic acid was used in all these treatments for the sole purpose of quenching positively charged holes remaining in the valence band of rutile. The role of ascorbic acid in promoting bacterial growth was expected to be minimal, as bacterial growth was not stimulated beyond that by the amount of Fe 2+ initially present in the m9K medium for the 'open-circuit' and dark controls. Even if there was any effect, this effect would have been present in all treatments and should not affect the relative comparison between them. ( b ) A significant positive correlation between the net growth of A. ferrooxidans in the reactor and net electric charge transferred from the P-chamber to the C-chamber ( P value <0.001). Full size image In contrast to the above treatments, maximal cell growth occurred when both rutile and visible light were present in the P-chamber. The photoelectrons generated in the P-chamber were spontaneously transported to the C-chamber owing to the potential difference between the two chambers. In the C-chamber, the photoelectrons reduced Fe 3+ to Fe 2+ , which was then oxidized by A. ferrooxidans to support its growth. In contrast to the experiment without rutile, the growth of A. ferrooxidans in the presence of rutile and light continued beyond 2.5 days, even when the Fe 2+ concentration remained low (~4,000 mg l −1 ). This sustained growth was ascribed to the regeneration effect of Fe 2+ from Fe 3+ reduction by photoelectrons as evidenced by a positive correlation between the net cell growth in the C-chamber and the number of photoelectrons transferred from the P-chamber to the C-chamber ( Fig. 2b ). In addition, photoelectrons significantly shortened the lag phase of A. ferrooxidans (compare the growth curves between 0 and 0.5 days, Fig. 2a ). Other semiconducting minerals, such as sphalerite ( Fig. 3a ) and goethite ( Fig. 3b ), showed a similar photocatalytic effect in promoting the growth of A. ferrooxidans . Significantly higher cell growth was observed in the presence of both the semiconducting mineral and visible light under the condition of a closed circuit than those under the other three conditions ( Fig. 3 ). 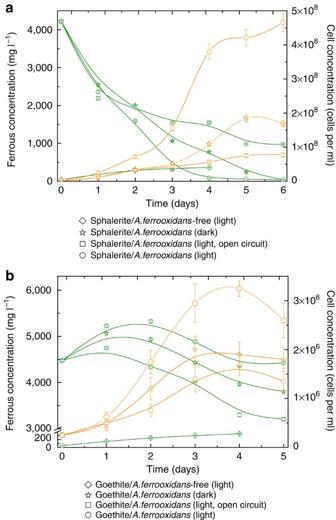Figure 3: Time course changes of Fe2+andA. ferrooxidansconcentrations using sphalerite or goethite as a semiconducting mineral under different conditions. The cathode electrolyte is either the m9K medium (experiments withA.ferrooxidans) or a modified Fe2+-free m9K medium (A.ferrooxidans-free experiments) by replacing 22.4 g l−1FeSO4·7H2O with 6.1 g l−1FeCl3(equivalent to 2.1 g l−1Fe3+conc.). The slightly lower Fe2+concentration at time zero (that is, 4,250 mg l−1in (b)) than the expected value from 22.4 g l−1FeSO4·7H2O (4,500 mg l−1) for the treatments withA.ferrooxidanswas probably due to oxidation of Fe2+and precipitation of ferric iron oxide. (a) In the presence of sphalerite in the P-chamber, photoelectrons reduced Fe3+, initially present in the modified m9K medium. When bacteria were added to the C-chamber in the dark, cell concentration increased (orange stars) using energy from the oxidation of Fe2+(green stars initially present in the m9K medium. In visible light, sphalerite photocatalysis occurred but when the circuit was open, cell concentration only reached 8.0×107cells ml−1(orange squares). In the presence of both sphalerite and cells, the photoelectrons stimulated the cell growth due to the continuous generation of Fe2+from the reduction of Fe3+by photoelectrons (orange and green circles for cell growth and Fe2+concentration, respectively). (b) In the presence of goethite, photoelectrons reduced Fe3+in the modified m9K medium. When bacteria were added to the C-chamber in the dark, cell concentration increased from 3.5×105cells ml−1to a maximum of 1.2×106cells ml−1(orange stars) by consuming energy released from the oxidation of Fe2+(green stars) present in the m9K medium. In visible light, goethite photocatalysis occurred but when the circuit was open, cell concentration only reached 5.1×105cells ml−1(orange squares), and the cell growth occurred at the expense of the m9K medium- Fe2+(green squares). In the presence of both goethite and cells, the photoelectrons stimulated the cell growth (orange and green circles for cell growth and Fe2+concentration, respectively). Figure 3: Time course changes of Fe 2+ and A. ferrooxidans concentrations using sphalerite or goethite as a semiconducting mineral under different conditions. The cathode electrolyte is either the m9K medium (experiments with A.ferrooxidans ) or a modified Fe 2+ -free m9K medium ( A.ferrooxidans -free experiments) by replacing 22.4 g l −1 FeSO 4 ·7H 2 O with 6.1 g l −1 FeCl 3 (equivalent to 2.1 g l −1 Fe 3+ conc.). The slightly lower Fe 2+ concentration at time zero (that is, 4,250 mg l −1 in ( b )) than the expected value from 22.4 g l −1 FeSO 4 ·7H 2 O (4,500 mg l −1 ) for the treatments with A.ferrooxidans was probably due to oxidation of Fe 2+ and precipitation of ferric iron oxide. ( a ) In the presence of sphalerite in the P-chamber, photoelectrons reduced Fe 3+ , initially present in the modified m9K medium. When bacteria were added to the C-chamber in the dark, cell concentration increased (orange stars) using energy from the oxidation of Fe 2+ (green stars initially present in the m9K medium. In visible light, sphalerite photocatalysis occurred but when the circuit was open, cell concentration only reached 8.0×10 7 cells ml −1 (orange squares). In the presence of both sphalerite and cells, the photoelectrons stimulated the cell growth due to the continuous generation of Fe 2+ from the reduction of Fe 3+ by photoelectrons (orange and green circles for cell growth and Fe 2+ concentration, respectively). ( b ) In the presence of goethite, photoelectrons reduced Fe 3+ in the modified m9K medium. When bacteria were added to the C-chamber in the dark, cell concentration increased from 3.5×10 5 cells ml −1 to a maximum of 1.2×10 6 cells ml −1 (orange stars) by consuming energy released from the oxidation of Fe 2+ (green stars) present in the m9K medium. In visible light, goethite photocatalysis occurred but when the circuit was open, cell concentration only reached 5.1×10 5 cells ml −1 (orange squares), and the cell growth occurred at the expense of the m9K medium- Fe 2+ (green squares). In the presence of both goethite and cells, the photoelectrons stimulated the cell growth (orange and green circles for cell growth and Fe 2+ concentration, respectively). Full size image The Fe 2+ concentration and cell growth profiles in the rutile-, sphalerite- and goethite-catalysed systems differed slightly under comparable experimental conditions. In the rutile-catalysed system, the Fe 2+ concentration was nearly constant in the first 0.5 day and then gradually decreased ( Fig. 2a ), indicating that the rate of Fe 2+ oxidation by A. ferrooxidans was initially equal to the rate of Fe 3+ reduction by photoelectrons, but the rate of Fe 2+ oxidation exceeded the rate of Fe 3+ reduction after 0.5 day, possibly because of the increased cell population. In contrast, in the sphalerite-catalysed system ( Fig. 3a ), the Fe 2+ concentration rapidly decreased, indicating that the rate of Fe 2+ oxidation by A. ferrooxidans well exceeded the rate of Fe 3+ reduction by photoelectrons. In the goethite-catalysed system, the Fe 2+ concentration initially increased (from 0 to 2 days, Fig. 3b ), implying that the rate of Fe 3+ reduction by photoelectrons was higher than the rate of Fe 2+ oxidation by A. ferrooxidans . After this period, cell growth seemed to enter the logarithmic phase, and the Fe 2+ concentration decreased owing to the increased rate of Fe 2+ consumption by A. ferrooxidans . In summary, these differences in the Fe 2+ concentration profiles and corresponding cell growth curves in the systems containing the three semiconducting minerals were ascribed to their respective different photovoltaic efficiencies. (see Supplementary Methods for the calculations of efficiencies). In the above three experiments involving rutile, sphalerite and goethite, the amounts of metal ions released from the minerals to solution and their effects on bacterial growth in the C-chamber were negligible. These minerals (40, 40 and 5–10 μm in average diameter) are not nanoparticles, and their solubilities are low [14] , [15] , [16] . The calculated soluble metal ion concentrations were 2.1 μg l −1 Ti 4+ for the rutile experiment, 23 μg l −1 Zn 2+ for the sphalerite experiment, and 54 μg l −1 Fe 3+ for the goethite experiment. Furthermore, if there were any effects from the trace amounts of soluble metals, they would have been the same for all treatments, and should not have influenced the relative differences in the bacterial growth yield between the controls (dark and open-circuit) and the treatments (with mineral and light under the closed circuit condition). The second experiment was designed to test the effect of light wavelength and intensity on the growth of the same bacterium ( Fig. 4 ). Five different wavelengths of visible light (420, 470, 520, 570 and 620 nm) with the same light intensity (8 mW cm −2 ) were chosen to study how A. ferrooxidans responded to rutile photocatalysis ( Fig. 4a ). The results clearly showed that, as light wavelength increased, bacterial concentration ( Fig. 4a ), the electron transfer rate (described as current density in Fig. 4b , that is, measured electric current per unit area of the rutile electrode), and the photoelectric efficiency ( Fig. 4c , orange curve) all decreased. The photoelectric efficiency profile closely matched the light absorption spectrum of rutile ( Fig. 4c , green curve). The calculated photoelectric efficiency for rutile (0.16–0.33%) was similar to the reported values of below 1% for commercial P25 TiO 2 powder under visible light [17] and 0.56% for dye-sensitized TiO 2 film under full sunlight [18] . Increasing light wavelength resulted in weaker optical absorption and lower photoelectric efficiency of rutile, which generated fewer photoelectrons and lower current density, and supported a lower amount of cell growth. Bacterial growth was also dependent on light intensity (light dosage). At a fixed wavelength (420 nm), after four days of incubation, cell concentration increased with increasing light intensity from 2 to 8 mW cm −2 ( Fig. 4d , red curve). On further increase to 16 mW cm −2 , cell concentration sharply decreased because of the low current density at this intensity ( Fig. 4d ). The cell concentration profile as a function of light intensity closely matched the current density profile ( Fig. 4d , green curve). 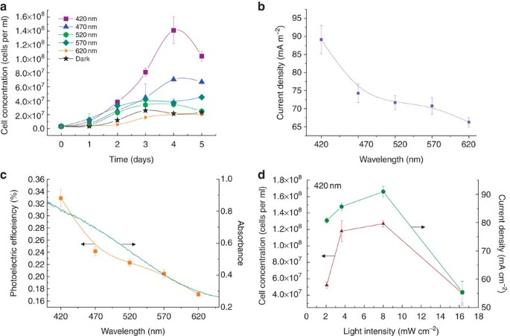Figure 4: Dependence ofA. ferrooxidansgrowth on light wavelength and intensity. (a) Growth curves ofA. ferrooxidansunder different conditions. This graph shows the dependence of cell growth on wavelength of visible light. A light intensity of 8 mW cm−2(of the rutile surface area) was used. (b) The dependence of current density on wavelength. The highest current density at 420 nm corresponds to the highest cell growth yield. (c) The photoelectric efficiency of the rutile-A. ferrooxidanssystem, as a function of light wavelength (orange curve), showing that the efficiency is the highest at 420 nm, which accounts for the highest cell growth yield. These measurements were made at a fixed light intensity 8 mW cm−2over the logarithmic phase of the cells. The light absorption spectrum of rutile is also plotted as a function of light wavelength (green curve). (d) The dependence of the cell concentration ofA. ferrooxidans(at day 4) on light intensity at a fixed wavelength of 420 nm (red curve). Current density is also plotted as a function of light intensity (green curve). Figure 4: Dependence of A. ferrooxidans growth on light wavelength and intensity. ( a ) Growth curves of A. ferrooxidans under different conditions. This graph shows the dependence of cell growth on wavelength of visible light. A light intensity of 8 mW cm −2 (of the rutile surface area) was used. ( b ) The dependence of current density on wavelength. The highest current density at 420 nm corresponds to the highest cell growth yield. ( c ) The photoelectric efficiency of the rutile- A. ferrooxidans system, as a function of light wavelength (orange curve), showing that the efficiency is the highest at 420 nm, which accounts for the highest cell growth yield. These measurements were made at a fixed light intensity 8 mW cm −2 over the logarithmic phase of the cells. The light absorption spectrum of rutile is also plotted as a function of light wavelength (green curve). ( d ) The dependence of the cell concentration of A. ferrooxidans (at day 4) on light intensity at a fixed wavelength of 420 nm (red curve). Current density is also plotted as a function of light intensity (green curve). Full size image In summary, these experiments demonstrated that mineral photocatalysis was light-dependent in a dose-dependent manner and that the spectrum of light-induced bacterial growth closely matched the light absorption spectrum of the minerals. The results showed different photon-to-biomass conversion efficiencies from the three semiconducting minerals (rutile, sphalerite and goethite), ranging from 0.13 to 0.18‰ for the rutile- A. ferrooxidans system to 0.25–1.9‰ for the sphalerite- A. ferrooxidans system. In comparison, the energy efficiency of photosynthesis, defined as the energy content of biomass that can be harvested annually divided by the annual solar irradiation over the same area, does not exceed 10‰ for crop plants, although short-term measurements can be higher [19] . In this study, the biomass conversion efficiencies were calculated based on energy flux from specific wavelengths instead of the full solar spectrum; therefore, the calculated conversion efficiencies in our system is not directly comparable to the value from photosynthesis [19] . Nonetheless, we presume the light-induced and mineral-mediated pathway for light-derived microbial growth is probably less efficient than photosynthesis. Growth of A. faecalis on photoelectrons Photoelectrons from the semiconducting minerals in the P-chamber also supported the growth of heterotrophic bacterium, A. faecalis , one of the most prevalent species of bacteria in natural soils [20] . In the presence of a simulated sun light source (Xe-lamp), photoelectrons from rutile in the P-chamber flew to the C-chamber, generating a higher current than that in the dark ( Fig. 5 ). Higher current in the light experiment significantly stimulated the growth of A. faecalis on the graphite electrode of the C-chamber, as revealed by the environmental scanning electron microscope (ESEM) images ( Fig. 6 ). Compared to the sparse distribution of a few short rod-shaped bacteria on the electrode surface in the dark ( Fig. 6b ), the light promoted the attachment of numerous rod-shaped bacteria to the electrode surface to form a visible biofilm ( Fig. 6a ). Quantitative analyses indicated that colony-forming units (CFU) in the presence of light (3×10 6 CFU cm −2 of the electrode area) were three orders of magnitude higher than that in the dark (2×10 3 CFU cm −2 ), where the initial cell concentration in the C-chamber was 8.3×10 7 ml −1 of the soil extract. These observations suggest that A. faecalis responded to photoelectrons and its growth was substantially stimulated by photoelectrons. 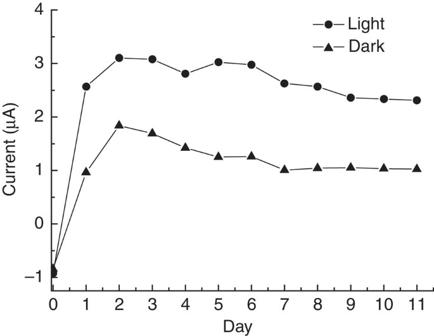Figure 5: Variations of electric current with time in the light and in the dark. The semiconducting mineral in the P-chamber is rutile, and the bacterium in the C-chamber isA. faecalisin soil extract. Light was provided with wavelength of 380–760 nm and an intensity of ~13.5 mW cm−2. The presence of electric current under the dark condition is inferred to be due to naturally present redox couples in soil extract. Figure 5: Variations of electric current with time in the light and in the dark. The semiconducting mineral in the P-chamber is rutile, and the bacterium in the C-chamber is A. faecalis in soil extract. Light was provided with wavelength of 380–760 nm and an intensity of ~13.5 mW cm −2 . The presence of electric current under the dark condition is inferred to be due to naturally present redox couples in soil extract. 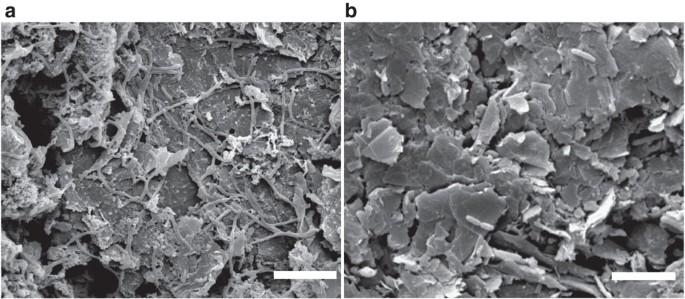Figure 6: Environmental scanning electron micrograph images ofA. faecaliscells on the cathode surface after 20 days of growth. (a) In the light (continuous wavelength 380–760 nm and intensity of ~13.5 mW cm−2) and (b) in the dark. The semiconducting mineral in the P-chamber is rutile, and the bacterium in the C-chamber isA. faecalisin soil extract. Scale bar, 5 μm. Full size image Figure 6: Environmental scanning electron micrograph images of A. faecalis cells on the cathode surface after 20 days of growth. ( a ) In the light (continuous wavelength 380–760 nm and intensity of ~13.5 mW cm −2 ) and ( b ) in the dark. The semiconducting mineral in the P-chamber is rutile, and the bacterium in the C-chamber is A. faecalis in soil extract. Scale bar, 5 μm. Full size image Response of a natural bacterial community to photoelectrons To confirm the occurrence of mineral photocatalysis-induced microbial metabolism in nature, the photoresponse of a natural bacterial community in a soil sample collected from Southern China was tested. This soil contained both natural microbes and semiconducting minerals (dominantly goethite). In these experiments, the process of photoelectron generation was simulated by setting a potential of −0.2 V (the amount of potential produced in a typical light experiment) to the electrode in the C-chamber. In the treatment with no applied voltage, electric current steadily decreased from 4 μA to around 0 μA in 5 days and stabilized at 0 μA ( Fig. 7 ). In contrast, the experiment with applied voltage produced a higher current for a longer time period: the current decreased from 2100 μA to around 850 μA by day 5, and stabilized at 850 μA afterwards ( Fig. 7 ). Phylogenetic analysis based on the 16S ribosomal RNA gene indicated that the bacterial community in the natural soil sample (at day 0) was diverse (Shannon index, 3.7, Simpson index, 27.4, Pielou evenness, 0.8, OTU number, 68) and consisted of Beta- and Gamma- subgroups of Proteobacteria, Bacteroidetes, Actinobacteria, and Acidobacteria ( Supplementary Fig. S1 ). The only clone sequence possibly related to a phototrophic bacterium was SZS′-0_77, but the DNA sequence was ~10% different from the closest representative sequence in NCBI, an uncultured Chloroflexi bacterium clone Tik_05 (AM749752). In the treatment with no applied voltage, the overall diversity remained high with time; also Pseudomonas and Pedobacter groups became enriched in the C-chamber over time. In contrast, in the treatment with applied voltage, the Chitinophaga , Pseudomonas , Alcaligenes and Pedobacter groups became enriched by day 5. By day 10, the Alcaligenes species constituted greater than 70% of the total bacterial population, in marked contrast to <8% in the control with no voltage ( Fig. 7 ). The application of voltage dramatically decreased the bacterial diversity as shown by both the OTU number and diversity indices, such as Shannon's index ( Supplementary Table S1 ). The observed correlation between electric current and the shift in the microbial community structure demonstrated that photoelectrons probably led to the enrichment and growth of certain heterotrophic bacteria such as Alcaligenes . Because of the lack of phototrophs in the soil sample and the absence of sunlight throughout the experiments (using applied voltage instead), interference from phototrophs was ruled out. 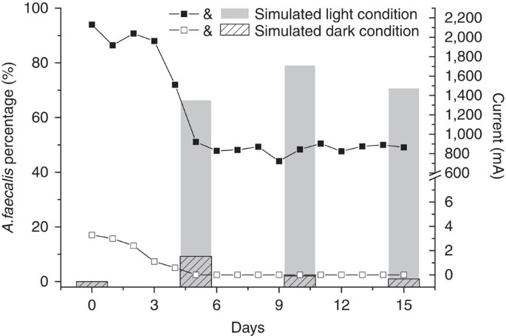Figure 7: Variation of electric current in a natural soil–water system and the corresponding change of the relative percentage ofA. faecalis. In this system, sterile soil extract was used as electrolyte in both chambers, and the natural red soil was added into the C-chamber. A −0.2 V (versus saturated calomel electrode) potential was applied on the electrode in the C-chamber to simulate the light condition, while the electrode with no applied voltage simulated the dark condition. The open and solid squares correspond to electric current values. The height of column represented the relative percentage ofA. faecalis. In the simulated light condition, the relative proportion ofA. faecalisbecame enriched (filled columns) over 15 days, whereas it slightly decreased (hatched columns near the bottom) in the simulated dark condition. Figure 7: Variation of electric current in a natural soil–water system and the corresponding change of the relative percentage of A . faecalis . In this system, sterile soil extract was used as electrolyte in both chambers, and the natural red soil was added into the C-chamber. A −0.2 V (versus saturated calomel electrode) potential was applied on the electrode in the C-chamber to simulate the light condition, while the electrode with no applied voltage simulated the dark condition. The open and solid squares correspond to electric current values. The height of column represented the relative percentage of A. faecalis . In the simulated light condition, the relative proportion of A. faecalis became enriched (filled columns) over 15 days, whereas it slightly decreased (hatched columns near the bottom) in the simulated dark condition. Full size image A. faecalis has versatile functions including degradation of polyaromatic hydrocarbons [21] and plastics [22] , arsenite oxidation [23] , heterotrophic nitrification-aerobic denitrification to remove ammonium in wastewater [24] , siderophore production, and promotion of plant growth in the soil rhizosphere [25] . In the presence of the semiconducting mineral CdS and light, NAD can be photoreduced to NADH via the direct electron transport from CdS to the enzyme transport chain of an Alcaligenes species [26] . The reducing power of NADH has been observed to support the growth of heterotrophic bacteria such as Escherichia coli [27] . Although the exact biochemical pathway of the photocatalyzed microbial growth is yet to be determined, it is likely that a similar mechanism may be responsible for the progressive enrichment of A. faecalis in the soil sample as a result of the photocatalysis by semiconducting minerals. Our results demonstrated an effect of the photocatalytic process on the growth of various bacteria. These results are in contrast to those previously reported about photocatalytic disinfection of bacteria by semiconductors, such as TiO 2 -based photocatalysts [28] . In those photocatalysts, photogenerated reactive oxygen species (ROS) were believed to be the 'killers' of bacteria, where the cell wall of bacteria adsorbed onto semiconductors could be quickly damaged by ROS through photocatalytic oxidation reactions [29] , [30] . Because of the short lifetime of ROS, only those microorganisms with an immediate contact with semiconductors are threatened [31] . However, to date, there is no research showing if photogenerated electrons can kill microorganisms. Spatial separation of the semiconducting minerals and the bacteria in our design would minimize any chance of damage to the bacteria by ROS, and, instead, photoelectrons would actually sustain microbial growth. Our data actually provided such evidence that the growth of non-phototrophic microorganisms could be stimulated by solar energy through the photocatalysis of semiconducting minerals. Photoelectrons generated by mineral photocatalysis are transferred across a relatively long distance through a conducting matrix to sustain the growth of non-phototrophic microorganisms. The results from this study were relevant to natural processes because our experimental system simulated the natural environment. The semiconducting minerals, such as oxides and sulfides used in this study, commonly exist on Earth's surface [32] , [33] . Autotrophic, heterotrophic, and soil bacterial communities are all ubiquitous in nature. Compounds of reducing potentials, such as ascorbic acid, humic acid and sulfides, are formed by decomposition of biomass or dissolution of minerals and are widespread in nature [32] , [34] , [35] . They can all serve as scavengers of positively charged holes [36] , [37] , [38] generated during mineral photocatalysis. The conductive wire, used in this study, is analogous to proteins and other cellular structures that facilitate transcellular electron transfer, such as the recently identified bacterial nanowires [39] . Non-phototrophic autotrophs and heterotrophs exist in abundance in both ancient and modern environments [40] , [41] . On early anoxic Earth, metal sulfide photocatalysis might have provided an energy-yielding pathway to support microbial growth. Once the atmosphere became oxygenated owing to the emergence of photosynthesis, mineral photocatalysis by Fe and Mn oxides could have supported various metabolic pathways such as sulfate reduction, nitrate reduction and iron oxidation. Our data demonstrate that the aerobic denitrifying ( A. faecalis ) and iron-oxidizing ( A. ferrooxidans ) bacteria can grow on energy released from photocatalysis of sulfides and oxides. In the modern environment, non-phototrophic microorganisms have been found in a number of extreme environments ranging from the driest desert [42] to the most acidic environments [43] , [44] . In these environments, organic matter is scarce and is generally produced by a subset of microorganisms such as chemolithotrophs [44] . The abundant existence of semiconducting minerals such as metal sulfides and oxides in the same environments [43] , [44] can produce photoelectrons through photocatalysis, which might have indirectly or directly fuelled non-phototrophic microorganisms, such as A. ferrooxidans and A. faecalis . Experimental configuration The experimental system used to investigate the role of semiconducting minerals in mediating the transfer of photoelectrons to bacteria had a dual-chambered design ( Fig. 1 ). The left chamber was for the photocatalytic reaction (P-chamber) and the right chamber was for the bioelectrochemical reaction (C-chamber). Each chamber was made of glass and had a volume of 350 ml. A glass tube (19 cm in length and 3 cm in inner diameter) connected the two chambers with a proton exchange membrane (Dupont, USA). Both chambers were sealed with a rubber septa. Unless otherwise specified, the P-chamber contained a natural mineral-coated electrode that was fabricated using a three-step procedure: mixing 0.54 g of mineral (rutile, sphalerite or goethite) powder and 0.06 g of acetylene black in an agate mortar until a homogeneous powder was obtained; adding ~0.3 ml. of polytetrafluoroethylene with a few drops of ethanol into the above mineral power until the mixture was solidified into gel; smearing the gel onto a graphite electrode (Hongfeng Carbon, Shanghai, China) (5×7 cm 2 in area and 5 mm in thickness) to form a thin mineral film of ~0.2 mm in thickness followed by air drying for 12 h at room temperature. The mineral-coated graphite electrode in the P-chamber and the graphite electrode in the C-chamber were externally connected with a copper wire to allow the electron transfer and the calculation of electric current by measuring voltage across a resistor ( Fig. 1 ). The glass wall of the P-chamber faced the light source and served as the only light-transmitting component of the device. A 300-W Xe lamp with a UV filter (Trusttech, China, irradiation wavelength 380–760 nm, light intensity 13.5 mW cm −2 ) was used as a visible light source. To minimize any heating effect of the lamp, an infrared filter was inserted in the light path to prevent any transmission of infrared light. The temperature of the solutions in both chambers was continuously monitored and it was nearly constant at 30 (±1) °C throughout all the experiments. A monochromator was used to obtain discrete wavelengths at 420, 470, 520, 570 and 620 nm. The distance between the light and the mineral-coated electrode was ~11 cm, but also adjustable to vary light intensity. An inlet of 1.7 mm in diameter in the rubber lid of the C-chamber allowed diffusion of ambient sterile O 2 and CO 2 into the chamber. The chemical reductant ascorbic acid (12.5 g l −1 ) in electrolyte KCl (2.5 g l −1 ) served as the scavenger of positively charged holes in the P-chamber. Unless specially stated, the C-chamber contained various mixtures including: Fe 3+ and/or Fe 2+ solutions in the m9K medium [45] (see below for its specific composition); a Fe 3+ /Fe 2+ solution containing A. ferrooxidans in the m9K medium; Luria-Bertani medium containing A. faecalis ; and a red soil slurry in sterile soil extract as an electrolyte. One modification was made to the m9K medium for the sphalerite/goethite experiments. Instead of 41.7 g l −1 FeSO 4 ·7H 2 O in the standard m9K medium used for the rutile experiments, 22.4 g l −1 FeSO 4 ·7H 2 O (that is, 4,500 mg l −1 Fe 2+ ) was used to make up the m9K medium for the sphalerite/goethite experiments. The whole system was placed on a magnetic stirrer (Tongji Instruments, Jiangsu, China) at a constant temperature of 30 °C. In the experiment involving the growth of the natural microbial community in the soil sample, to accelerate the generation of photoelectrons, an external voltage was applied on the C-chamber with a CHI model 660 °C potentiostat (Shanghai Chenhua Instruments Corporation, China) using a conventional three-electrode system. In this system, the cathode in the C-chamber was set as a working electrode and the anode in the P-chamber as a counter electrode. The reference electrode was a saturated calomel electrode (SCE, 0.242 V corrected to a normal hydrogen electrode (NHE)), which was placed close to the working electrode. Bacterial culture conditions and experimental treatments A strain of A. ferrooxidans was isolated from water samples collected from an acid pit in Shanxi Province, China. The water samples showed a brown-black colour and pH of 2.2. A modified 9K medium (hereafter referred to as the m9K medium) (0.15 g l −1 (NH 4 ) 2 SO 4 , 0.05 g l −1 KH 2 PO 4 , 0.05 g l −1 KCl, 0.5 g l −1 MgSO 4 ·7H 2 O, 0.01 g l −1 Ca(NO 3 ) 2 ·4H 2 O, 41.7 g l −1 FeSO 4 ·7H 2 O) [45] was used for isolation of A. ferrooxidans (see Supplementary Methods for the isolation procedure). This isolate was identified as A. ferrooxidans (100% similarity) by sequencing the nearly full length of the 16S rRNA gene (GenBank accession number HQ603786 ). A. ferrooxidans was inoculated to the C-chamber at 3.5×10 5 cell ml −1 (final conc., inoculation ratio: 10% V/V) for all experiments involving this strain. Four treatments were set up: the P-chamber contained a mineral-coated graphite anode with light irradiation; the C-chamber contained the Fe 2+ -free m9K medium that was supplemented with Fe 3+ (as FeCl 3 at 6.1 g l −1 ) without any cells. This experiment was designed to test the production of photoelectrons from semiconducting minerals; The P-chamber contained mineral-coated graphite anode without light and the C-chamber contained cells; the P-chamber contained a graphite anode without mineral-coating but with light; the C-chamber contained the m9K medium and A. ferrooxidans cells; and the P-chamber contained mineral-coated graphite anode with light irradiation, whereas the C-chamber contained the m9K medium and A. ferrooxida ns. A strain of A. faecalis (ATCC 8750) was purchased from the Chinese General Microbiological Culture Collection Center at the Institute of Microbiology, Chinese Academy of Sciences in Beijing. Cells grown to the logarithmic phase (see Supplementary Methods for the culturing procedure) were transferred to a culture medium with a diluted nutrient broth (25%) in the C-chamber at time zero. The growth of A. faecalis was monitored under light and dark conditions with rutile as a semiconducting mineral. A soil sample was collected from a field site in southern China. Sterile and non-sterile extracts were obtained (see Supplementary Methods for the details of the acquisition of soil extracts) and used as electrolyte in the P- and C-chamber, respectively. Bacterial diversity in the C-chamber was monitored over a 15-day period. Analytical techniques The bacterial population density was determined by either direct counting ( A. ferrooxidans ) or colony forming units (CFU) ( A. faecalis ) (see Supplementary Methods for details). The ferrous concentration was determined spectrophotometrically with the o -phenanthroline method [46] by using an Agilent HP8453 spectrophotometer. The irradiation intensity of the Xe lamp was adjustable and measured by using an irradiation meter (Beijing Normal University Instruments, Beijing, China). Current density from the P-chamber to the C-chamber ( Fig. 4 ) was calculated by integrating the current-time curves (see Supplementary Methods for details). The growth of A. faecalis cells was visually observed by using a FEI Quanta 200FEG ESEM at ×5,000 magnification. Before the observation, a small piece of the graphite electrode (in the C-chamber) was scraped off. The cells on the graphite electrode were fixed using 2.5% glutaraldehyde at 4 °C overnight and washed with 0.1 M sodium phosphate buffer (pH 7.2) 3 times (each for 15 min). The cells were dehydrated with a series of ethanol-water mixtures (30, 50, 70, 85, 95 and 100 vol% of ethanol) for 15 min each. After critical point drying, the samples were mounted on a silicon plate using double-sided carbon tape and then coated with gold for ESEM observation. Calculation of the energy conversion efficiencies The photoelectric efficiency was calculated by dividing the number of photoelectrons flowing from the P-chamber to the C-chamber by the number of photons received on the rutile surface over the logarithmic growth period of the A. ferrooxidans . Two methods were used to calculate the photon-biomass conversion efficiency. In the first method, the efficiency was calculated by dividing the amount of energy derived from Fe 2+ oxidation in the C-chamber (that is, the energy output to support the growth of A. ferrooxidans ) by the amount of light energy received in the P-chamber (that is, energy input) over the logarithmic growth period (1.5 to 4 days, Fig. 2 ). In the second method, the efficiency was calculated by dividing the amount of energy required to result in the observed cell growth by the amount of light energy received in the P-chamber (see Supplementary Methods for examples for each method). Molecular microbiological techniques Genomic DNA was extracted from 7 samples including the original soil sample and day 5, 10 and 15 samples from both light and dark treatments according to previously reported procedures [47] , [48] (See Supplementary Methods for details). Terminal restriction fragment length polymorphism analysis was carried out for all seven samples, and the Shannon index (H), Simpson index (D), and Pielou evenness (J) were calculated based on the relative peak area. The relative proportion of A. faecalis was estimated from the area of the peak belonging to this strain relative to the total area of all the peaks in the terminal restriction fragment length polymorphism profiles. Two bacterial 16S rRNA gene clone libraries were constructed from the seven samples: one for the natural soil sample (SZS′-0) and the other for the 15-day soil sample from the C-chamber with a bias voltage (SZS′-1). A total of180 and 190 positive clones were picked from SZS′-0 and SZS′-1 clone libraries, respectively and representative clones were sequenced. The nucleotide sequences determined have been deposited in the GenBank database under accession numbers: HM049659 - HM049712 . How to cite this article: Lu, A. et al . Growth of non-phototrophic microorganisms using solar energy through mineral photocatalysis. Nat. Commun. 3:768 doi: 10.1038/ncomms1768 (2012).